Tyrosine-mediated two-dimensional peptide assembly and its role as a bio-inspired catalytic scaffold In two-dimensional interfacial assemblies, there is an interplay between molecular ordering and interface geometry, which determines the final morphology and order of entire systems. Here we present the interfacial phenomenon of spontaneous facet formation in a water droplet driven by designed peptide assembly. The identified peptides can flatten the rounded top of a hemispherical droplet into a plane by forming a macroscopic two-dimensional crystal structure. Such ordering is driven by the folding geometry of the peptide, interactions of tyrosine and crosslinked stabilization by cysteine. We discover the key sequence motifs and folding structures and study their sequence-specific assembly. The well-ordered, densely packed, redox-active tyrosine units in the YYACAYY (H-Tyr-Tyr-Ala-Cys-Ala-Tyr-Tyr-OH) film can trigger or enhance chemical/electrochemical reactions, and can potentially serve as a platform to fabricate a molecularly tunable, self-repairable, flat peptide or hybrid film. A cellular membrane can modify its local shape partly via a protein-involved organizing process [1] . For example, clathrin forms an intricate assembly on the membrane, leading to endocytosis, by framing the high curvature of budding vesicles [2] . The SNARE complex brings two opposing lipid bilayers in proximity to induce membrane fusion and changes in curvature [3] . Such dynamic remodelling by proteins suggests new possibilities for multifunctional and programmable interfaces that can respond by changing their shape in response to environmental stimuli. However, with regard to synthetic systems, it has been an ongoing challenge to understand the precise mechanism of dynamic morphology changes at the molecular level and develop a new strategy for intelligent material applications based on rational sequence design. There is a continuous interplay between the two-dimensional (2D) crystal lattice structure and the geometry of the interface on which it is placed [4] . As the elastic-bending energy is high in most cases, the overall shape of the two-dimensionally assembled structure follows the shape of the interface. In addition, at the microscopic level, 2D ordering on a curved surface typically generates topological defects [5] , [6] , [7] , [8] , [9] , such as disinclination and dislocation, or induces symmetry-breaking instability [10] because the local ordering favoured by molecular interactions cannot propagate laterally throughout an entire system on a curved surface. For example, hexagonally close packing of spherical particles cannot perfectly tile a curved surface without heptagonal or pentagonal packing [6] , [7] , [8] . The geometric constraint imposed by curvature, nevertheless, can be overcome, and planar facets can appear when the elastic modulus of a 2D crystal is sufficiently large or the interfacial tension is weak. For example, faceted surfaces can be found in viral capsids formed by the crystalline packing of proteins [11] , hydrophobin protein film [12] , vesicles assembled from block copolymers [13] , wax colloidal disks packed with surfactants [14] or smectic A droplet on a flat substrate [15] . Faceting is a fascinating example to demonstrate how the balance between interface tension and molecular ordering controls morphology. To the best our knowledge, however, faceted morphology has never been observed in peptide assembly. The films composed of currently available peptide sequences do not have a sufficiently high elastic modulus to overcome the elastic-bending energy of the droplet. In this study, we develop a peptide-based, sequence-specific method that allows for the precise tuning of molecular structures, site-selective functionalization and control of intermolecular force. As a result, the assembly process is controllable in an entire droplet, flattening the rounded top into a plane by forming a macroscopic 2D crystal structure, and this is scalable to a large length (>100 cm 2 ; Fig. 1d ; Supplementary Fig. 1 ). 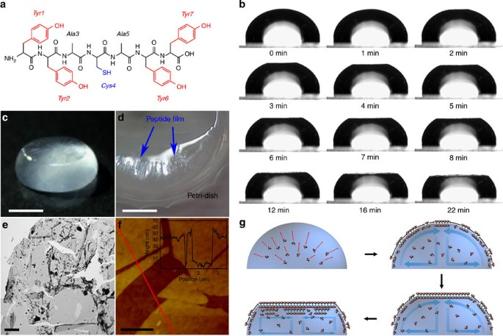Figure 1: Facet formation of water droplets by 2D peptide films. (a) Chemical structure of YYACAYY. (b) Optical microscopy images of a water droplet at different incubation times. The shape evolution of the droplet was monitored from a side view. A bright region in the middle of a droplet is due to the backlight transmission. (c) An oblique view of the droplet with a single large facet. A sharp boundary of the facet edge was observed. (d) A large and thick peptide film formed on the whole air/water interface in a Petri dish. For this camera image, the 5-ml of YYACAYY peptide solution was transferred to a Petri dish. (e,f) TEM (e) and AFM (f) image of large 2D films formed from 1 mg ml−1peptide solution (1.1 mM). (g) Schematics of the facet-forming mechanism with the YYACAYY solution. YYACAYY peptides float on air/water interface, and they are assembled into the peptide rafts at various positions on the surface. The peptide rafts migrate forwards top of the droplet, which results in the growth of the film and leads to facet formation. Scale bar, 0.5 cm (c), 1 cm (d), 5 μm (e), 1 μm (f). Figure 1: Facet formation of water droplets by 2D peptide films. ( a ) Chemical structure of YYACAYY. ( b ) Optical microscopy images of a water droplet at different incubation times. The shape evolution of the droplet was monitored from a side view. A bright region in the middle of a droplet is due to the backlight transmission. ( c ) An oblique view of the droplet with a single large facet. A sharp boundary of the facet edge was observed. ( d ) A large and thick peptide film formed on the whole air/water interface in a Petri dish. For this camera image, the 5-ml of YYACAYY peptide solution was transferred to a Petri dish. ( e , f ) TEM ( e ) and AFM ( f ) image of large 2D films formed from 1 mg ml −1 peptide solution (1.1 mM). ( g ) Schematics of the facet-forming mechanism with the YYACAYY solution. YYACAYY peptides float on air/water interface, and they are assembled into the peptide rafts at various positions on the surface. The peptide rafts migrate forwards top of the droplet, which results in the growth of the film and leads to facet formation. Scale bar, 0.5 cm ( c ), 1 cm ( d ), 5 μm ( e ), 1 μm ( f ). Full size image Faceting of water droplet by peptide assembly One advantage of peptide-based approaches is the ability to encode necessary information to address geometrical parameters and control the physical/chemical properties of the assembled structure [16] , [17] , [18] , [19] . By designing sequences, three-dimensional folding can be controlled, and various intermolecular forces to drive the assembly can also be directed at the atomic level. Various peptides and their derivatives have been identified as achieving interesting hierarchical architectures, including tubes [20] , [21] , [22] , [23] , [24] , fibres [25] , [26] , [27] , [28] , planar films [29] , [30] , [31] , [32] , [33] , ribbons [26] , [34] and three-dimensional networks [35] , [36] , [37] , [38] , [39] . We systematically introduced repeating tyrosine units into peptides of various lengths to study the impact of the peptide sequence on self-assembly. Tyrosine has a redox-active phenolic group, which can affect folding geometry dynamically [40] and facilitate proton-mediated electron transport [41] . We investigated the sheet-forming propensity of all possible 7-mer sequence domains occurring in an amyloidogenic protein, β 2 -microglobulin, and discovered an important role of the tyrosine-rich regions ( Supplementary Fig. 2 ). In a family of elastic proteins, such as resilin [42] and gluten [43] , the chemical crosslinks between tyrosine residues induce a protein network, providing high elastic modulus and efficient energy storage. Cysteine was also tested with regard to conferring folding stability through disulphide bridges [44] . We inserted alanine and phenylalanine at specific sites along the peptide chain to evaluate their self-assembly mechanism. Table 1 lists all 17 sequences that were classified according to their macroscopic behaviour. Table 1 Summary of peptides studied for the assembly. Full size table The arrangement of each amino acid and its composition were the main determinants of the peptide nanostructures ( Table 1 ). The detailed rationale for the sequence design was described in Supplementary Table 1 . The peptides were dissolved in 50 mM HEPES buffer (pH 7.4) and placed on siliconized glass. All transmission electron microscopy (TEM) images of the resulting structures are shown in Supplementary Fig. 3 . Dityrosine (YY) and trityrosine (YYY) formed long nanofibres that were 15 nm in diameter in aqueous solution, whereas the more hydrophobic tetratyrosine (YYYY) tended to bundle into random aggregates. CYY formed fibres, YCY and CYYCYYC aggregated randomly. However, we observed a faceting phenomenon in several sequences that were symmetric and had cysteine at the centre. YYCYY was the first sequence in our study that was found to form a facet within 10 min under our experimental conditions ( Supplementary Fig. 4 ). While searching for other sequences, we found that facets were formed within 1 min when alanines were inserted between cysteine and tyrosine (YYACAYY), representing the highest facet-forming capability and highest quality. Among the eight sequences that formed facets, YYACAYY was chosen in this study to describe the detailed mechanism. The faceting of a water droplet by YYACAYY could be clearly observed with the naked eye, and its kinetics and behaviour were monitored using optical camera side view observations ( Fig. 1a and Supplementary Movie 1 ). Under typical conditions, the volume of the YYACAYY solution was 80 μl, but this volume was scalable to larger volumes. For example, facets could be formed in a 5-ml droplet and the large film can form on a Petri dish ( Fig. 1d ). Closer observation revealed that the faceting began in the centre of the droplet within 1–2 min and grew continuously in the lateral direction. This lateral growth stopped after ~20 min when the size of the facet was close to the circumference of the water/glass boundary. The facet formation exhibited self-repairing properties ( Supplementary Fig. 5a and Supplementary Movie 2 ), and defects or cracks introduced intentionally by a needle were also repaired spontaneously ( Supplementary Fig. 5b ). Facet formation was observed at a wide range of pH (between 3 and 8), but the kinetic activity was the highest at pH 5.5, which is close to the isoelectric point of YYACAYY ( Supplementary Fig. 6 ). Facets were formed more quickly at 4 °C than at room temperature or at 60 °C. As facet formation needed to overcome the elastic-bending energy of the water droplet, the facet-forming kinetics became much slower for a droplet with a high curvature. When a droplet was placed on a hydrophobic Teflon surface, the curvature increased at the given volume. As a result, the facet formed more slowly, with a smaller final facet size ( Supplementary Fig. 7 ). The facet-forming kinetics also depended on the size and initial curvature of the droplet ( Supplementary Fig. 8 ). Faceting was the result of peptide film assembly at the air/water interface, as shown by TEM analysis ( Fig. 1e ), atomic force microscopy (AFM; Fig. 1f ) and fluorescence imaging ( Supplementary Fig. 9 ). The films at the air/water interface ( Fig. 1b ) were carefully transferred to a silicon substrate or carbon grid and washed with distilled water to remove the salts for clear images. The AFM data showed that the film was very flat and uniform ( Fig. 1f and Supplementary Fig. 10 ). The TEM images ( Fig. 1e and Supplementary Fig. 11 ) also showed uniform and laterally extended peptide films formed at the air/water interface. 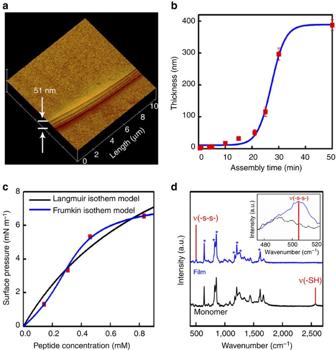Figure 2: Chemical and structural analysis of the peptide film. (a) AFM image showing that multiple nanosheets are stacked (20 min assembly,Z-range: 10 nm). (b) The plot of the thickening of a film as a function of assembly time. The error bars represent the standard deviations of the means of five independent determinations from two separate experiments. (c) Changes in the surface pressure with varying peptide concentration. The surface pressure at different concentrations was used with the saturated surface pressure shown in the surface pressure versus time plot (Supplementary Fig. 31a). The experimental data show a close fit to the Langmuir and Frumkin isotherm models. The Frumkin isotherm model (R2=0.998) fits better than the Langmuir isotherm model (R2=0.966). (d) Raman spectra of monomeric peptides (black line) and films (blue line). Tyrosine peaks are indicated with a star (*). The peak at 503 and 2,568 cm−1indicates disulphide (–S–S–) and sulfhydryl (–SH) group, respectively. The Raman signal over the range of 460–540 cm−1is enlarged (inset). Figure 2b shows how the thickness of the peptide film at the air/water interface evolves. The peptide films were originally thin but grew thicker over time. Figure 2: Chemical and structural analysis of the peptide film. ( a ) AFM image showing that multiple nanosheets are stacked (20 min assembly, Z -range: 10 nm). ( b ) The plot of the thickening of a film as a function of assembly time. The error bars represent the standard deviations of the means of five independent determinations from two separate experiments. ( c ) Changes in the surface pressure with varying peptide concentration. The surface pressure at different concentrations was used with the saturated surface pressure shown in the surface pressure versus time plot ( Supplementary Fig. 31a ). The experimental data show a close fit to the Langmuir and Frumkin isotherm models. The Frumkin isotherm model ( R 2 =0.998) fits better than the Langmuir isotherm model ( R 2 =0.966). ( d ) Raman spectra of monomeric peptides (black line) and films (blue line). Tyrosine peaks are indicated with a star (*). The peak at 503 and 2,568 cm −1 indicates disulphide (–S–S–) and sulfhydryl (–SH) group, respectively. The Raman signal over the range of 460–540 cm −1 is enlarged (inset). Full size image Structural analysis of peptide film Individual YYACAYY peptide films were composed of multiple vertically stacked thin nanosheets. AFM analysis along the film edges showed evidence of nanosheet stacking ( Fig. 2a and Supplementary Fig. 12 ) and a minimum thickness of 1.4 nm ( Supplementary Fig. 13 ); these 1.4 nm-thick nanosheets were also observed at an early stage of film growth at low peptide concentrations ( Supplementary Fig. 14 ). The minimal film formation concentration was 0.22 mM, but only small pieces of scattered, thin nanosheets were formed at this concentration. We believe that the 1.4-nm-thin sheets were formed initially and grew vertically into a thick film. Supplementary Fig. 12 shows a result from the multiple stacking of the thin nanosheets (1.4 nm). X-ray diffraction (XRD) analysis shows that the peptide film is crystalline ( Supplementary Fig. 15 ). As the peptide film is very thin, 80 films were multiply stacked and dried on a silicon substrate for the analysis. As shown in Supplementary Fig. 15 , the large, intense peak at 13.5 Å appears to be the result of the layer thickness, which is close to the typical 1.4 nm for the nanosheets. The size and thickness of the films increased as the peptide concentration increased ( Supplementary Fig. 10 ). An in situ observation of the droplet using fluorescence microscopy directly showed that raft-like nanosheets formed inside ( Supplementary Fig. 16 ) or on the droplet and subsequently migrated towards the top of the droplet, resulting in the flattening of the droplet by the peptide film ( Supplementary Fig. 17 ). The film formation was favoured on the curved surface over the flat surface. This observation implies that curvature-induced assembly was involved. As another factor, the convection inside the droplet and the different evaporation rate of water seem to contribute to the film formation ( Supplementary Movie 3 ). The flattening of the droplet indicates that the peptide film was stiff enough to overcome the surface pressure of the droplet. From the final shape of the flattened droplet ( Fig. 1b ), the elastic modulus of the peptide film can be calculated using finite element (FE) analysis by counter balancing the droplet deformation energy. In this analysis, the film size ( a ) and droplet size ( L ) were the measured values (5.1 and 6.5 mm, respectively) from Fig. 1b . The degree of bending ( h ) was calculated as a function of the elastic modulus of the peptide film. Here h indicates how much the central position of the flat peptide film was bent by the surface pressure ( P ), as defined in Fig. 3a . The simulated results ( Fig. 3b ) clearly confirmed that the degree of bending decreased significantly with the increase in the elastic modulus. Assuming that the bending becomes visible with naked eye when h is larger than 0.2 mm (~ two orders of magnitude of the film thickness), the elastic modulus of the flattened peptide films would be larger than 8 GPa. The nanoindentation analysis ( Supplementary Fig. 18 ; Supplementary Note 1 ) showed that the measured elastic modulus was 8.4 GPa. In addition, the final diameter ( a ) of the film could be predicted by setting the surface energy of the peptide film equal to the elastic-bending energy ( Fig. 3b,c ; Supplementary Fig. 19 ). As expected, the final film size was reduced as the droplet curvature became larger at a given elastic modulus. Similarly, the smaller film was formed with the smaller elastic modulus. These results are congruent with the experimental data. 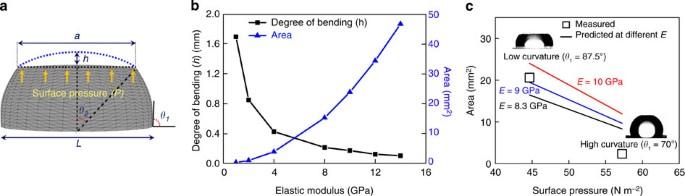Figure 3: Mechanical analysis of peptide film. (a) Schematic diagram for calculating the surface pressure of a droplet. For the droplet with low curvature (Fig. 1d), surface pressure (P),θ1,θ2,aandLwere measured as 44.65 N m−2, 87.5°, 42°, 5.1 mm, and 6.5 mm, respectively. (b) Changes in the degree of bending (h) and the final area of the film as a function of the elastic modulus. (c) Changes in the area of the peptide film with the surface pressure at various elastic modulus. On the basis of two droplets with low (Fig. 1b) and high (Supplementary Fig. 19) curvature, the surface pressure and the final areas were experimentally measured and were also pointed on the plot. For the droplet with high curvature,P,θ1,θ2,aandLwere 57.23 N m−2, 70°, 20°, 4.7 mm, and 1.7 mm, respectively. Figure 3: Mechanical analysis of peptide film. ( a ) Schematic diagram for calculating the surface pressure of a droplet. For the droplet with low curvature ( Fig. 1d ), surface pressure ( P ), θ 1 , θ 2 , a and L were measured as 44.65 N m −2 , 87.5°, 42°, 5.1 mm, and 6.5 mm, respectively. ( b ) Changes in the degree of bending ( h ) and the final area of the film as a function of the elastic modulus. ( c ) Changes in the area of the peptide film with the surface pressure at various elastic modulus. On the basis of two droplets with low ( Fig. 1b ) and high ( Supplementary Fig. 19 ) curvature, the surface pressure and the final areas were experimentally measured and were also pointed on the plot. For the droplet with high curvature, P , θ 1 , θ 2 , a and L were 57.23 N m −2 , 70°, 20°, 4.7 mm, and 1.7 mm, respectively. Full size image Role of peptide dimers in assembly To understand the assembly mechanism, we first analysed the peptide film using electrospray ionization (ESI) and matrix-assisted laser desorption/ionization (MALDI) mass spectrometry. Both analyses showed that the dimerization of YYACAYY occurred during film assembly ( Supplementary Figs 20 and 21 ). Raman spectra confirmed that this dimerization was due to disulphide bonding between two cysteines. A signal at 2,568 cm −1 (the –SH stretching vibration), which was observed in the peptide solution before assembly, disappeared after film formation, and a new signal appeared at 503 cm −1 , which corresponds to the S–S stretching frequency ( Fig. 2d and Supplementary Table 2 ). Additional evidence for disulphide bond formation included the disassociation of dimers into monomers with the addition of dithiothreitol (DTT; Supplementary Fig. 21 ). The films were broken when treated with 50 mM DTT for 30 min; the dimer peak observed with MALDI completely disappeared, and only the monomer peak was observed. The fact that adding β-mercaptoethanol decreased the faceting kinetics also demonstrated the importance of disulphide bonding in assembly ( Supplementary Fig. 22 ). As another evidence for the important role of dimers in film formation, we also observed that the film assembly kinetics depended on the concentration of the YYACAYY dimer. The incubation in dimethylsulphoxide (DMSO) solvent can convert the monomers to dimers as confirmed with HPLC data ( Supplementary Fig. 23 ) and Raman spectra ( Supplementary Fig. 24 ). The increase of dimer concentration and the intentional addition of pre-formed dimers can increase the kinetics of film formation significantly. From experiments with cysteine-replaced sequences, such as YYAEAYY and YYAKAYY, we verified that disulphide bonding is essential for peptide film formation and subsequent faceting. Although YYAEAYY and YYAKAYY can form much thinner films than YYACAYY, these motifs never produce a facet. We also observed that the facet did not occur even with YYACAYY in the oxygen-free desiccator. These results suggest that disulphide bridges are involved in film thickening and thus provide sufficient mechanical strength to overcome the elastic-bending energy. In addition to the disulphide-bridged dimerization, the conformation changes of the peptide were observed in the film based on Fourier transform infrared (FT-IR) analysis ( Supplementary Fig. 25 ). In particular, the bands at 3,148, 1,373, 1,240 and 1,172 cm −1 were decreased and red shifted, indicating that the electrons of the phenyl group were delocalized ( Supplementary Table 3 ). This result reflects π–π stacking between adjacent tyrosines during film formation. The increased peak intensities at 2,928, 2,868, 1,450 and 1,286 cm −1 indicated that the side chain of alanine residues and the peptide backbone were screened from the polar solvent when the peptides were aligned into an ordered architecture. Interestingly, the newly appeared peak at 1,657 cm −1 in deconvoluted FT-IR spectra ( Supplementary Fig. 26 ) showed that the peptide folded partially into α-helical conformation after the film formation. After finding that the dimerization of YYACAYY plays an important role in the assembly, possibly accompanied by the conformational change, we characterized in detail the conformational preferences of the monomers and the dimers in solution. The monomers could be separated from the as-prepared samples containing some dimers by prep-HPLC. The dimers can be made by an oxidative disulphide bond formation with the addition of DMSO. Molecular structure of peptides The detailed structures of the monomers and dimers were determined by 2D nuclear magnetic resonance (NMR) spectroscopy. The folding change from monomers to dimers could be monitored by the resonance assignment after 0, 24 and 48 h oxidation with DMSO. As shown in Fig. 4a , the monomeric YYACAYY displayed only sequential nuclear Overhauser effect (NOE) connectivities, implying that monomers do not exhibit any dominant folding. After 48 h, peptide was completely oxidized to the dimers, showing not only sequential NOE connectivities but also non-sequential connectivities characteristic of an α-helix, specifically d αN ( i , i +3), d βN ( i , i +3), d αN ( i , i +4) and d βN ( i , i +4) ( Fig. 4c ). The NOE connectivities of the YYACAYY dimer are summarized in Fig. 4d . It is interesting to note that the short peptide with only seven amino acids had connectivities between the residues Tyr1–Cys4, Tyr2–Ala5, Tyr2–Tyr6, Ala3–Tyr6 and Ala3–Tyr7. The amide protons temperature coefficient has been used to predict hydrogen bond donors. The values above −4.5 p.p.b. K −1 indicate that the amide proton is involved in intramolecular hydrogen bonding [45] . The amide protons temperature coefficients for Ala5 and Tyr6 at the end of helix region were −4.3 and −4.1 p.p.b. K −1 , respectively. The amide protons temperature coefficients of Tyr7 (−4.9 p.p.b. K −1 ) was above compared with those of other residues (below −6.0 p.p.b. K −1 ), implying that these amide protons formed stable hydrogen bonds. The amide protons of Tyr6 and Tyr7 remained for 24 h after 100 μl of D 2 O was added to the peptide for deuterium exchange with the amide protons, indicating that these amide protons formed stable hydrogen bonds ( Supplementary Fig. 27 ). A structure calculation of the peptide was carried out using the standard protocol of the Cyana2.1 program in a LINUX environment [46] . A total of 100 structures were calculated from a set of 49 NOEs comprising 26 sequential ( i−j =1) and 23 medium (2 ⩽ i−j ⩽ 4) or long-range ( i−j ⩾ 5) NOEs. As shown in Fig. 4f , the 20 lowest energy structures for the YYACAYY dimer showed that the occurrence of φ and ψ angles for all of the residues in the Ramachandran plots was 98.0% in the most favoured regions, which corresponds to the right-handed α-helix conformation. 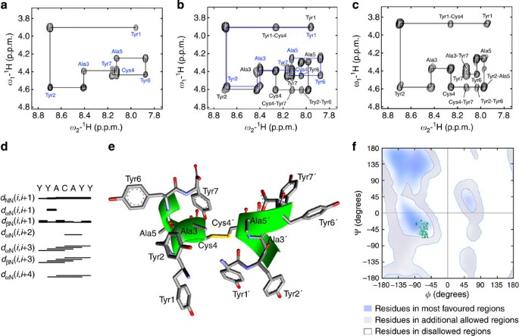Figure 4: NMR analysis of peptides. (a–c) Resonance assignments of YYACAYY peptide were analysed after 0 h (a), 24 h (b), 48 h (c) of adding DMSO for oxidative disulphide bond formation. In panelsa–c, resonance assignments of monomer and dimer are presented in blue- and black-line. They show that monomeric YYACAYY oxidizes to dimer with appearance of non-sequential NOE connectivities as incubation period increases. (d) Summary of NOE connectivities of dimer YYACAYY peptide. (e) Lowest energy NMR structure of dimeric peptide. The molecular structure are shown with a stick model where carbon, oxygen and nitrogen are presented in grey, red and purple, respectively. Helically coiled peptide backbones are visualized as a green ribbon. (f) Ramachandran plot of 20 lowest energy NMR structures for dimeric YYACAYY. Figure 4f shows that each monomer connected by the disulphide bond has the right-handed α-helical structure from Tyr2 to Tyr6. This equivalence resulted in 3.7 residues per turn and 5.5 Å as the pitch of the α-helix (the vertical distance between one consecutive turn of the helix). The height of the dimer was ~1.4 nm, measured from the distance between Tyr2 and Tyr6'. This result was close to the smallest thickness (1.4 nm) observed in the AFM analysis, which strongly suggests that the dimers acted as building blocks. It is also noteworthy that all phenolic ring groups in each monomer faced towards solvent. In the revealed dimer structure, the backbone structure was stabilized into a helix by the dimerization. The eight tyrosine groups were arranged along the vertical and lateral directions. Such folding geometry may help to facilitate the tyrosine-mediated interaction between dimers to be assembled into a continuous structure of stacked nanosheets. Figure 4: NMR analysis of peptides. ( a – c ) Resonance assignments of YYACAYY peptide were analysed after 0 h ( a ), 24 h ( b ), 48 h ( c ) of adding DMSO for oxidative disulphide bond formation. In panels a – c , resonance assignments of monomer and dimer are presented in blue- and black-line. They show that monomeric YYACAYY oxidizes to dimer with appearance of non-sequential NOE connectivities as incubation period increases. ( d ) Summary of NOE connectivities of dimer YYACAYY peptide. ( e ) Lowest energy NMR structure of dimeric peptide. The molecular structure are shown with a stick model where carbon, oxygen and nitrogen are presented in grey, red and purple, respectively. Helically coiled peptide backbones are visualized as a green ribbon. ( f ) Ramachandran plot of 20 lowest energy NMR structures for dimeric YYACAYY. Full size image The circular dichroism (CD) spectra in aqueous solution provide the additional evidence that the YYACAYY dimers have a high tendency to form a right-handed α-helix. The optical rotatory properties of poly- L -tyrosine or tyrosine-rich peptide (TRP) have been reported to be very different from those of common peptides [47] , [48] , [49] , [50] , [51] , [52] , [53] , [54] . A TRP with a right-handed α-helical conformation has four π–π* side-chain transitions (analogous to the A 1g , B 1u , B 2u and E 1u states of benzene) at about 200, 230 and 280 nm in neutral aqueous solution [51] , [52] , [53] . Around 200 nm, mixing the amide π–π* transition and two π–π* transitions of phenolic side chain produced a strong positive peak, as shown in the CD spectra of YYACAYY peptide [53] . Similar to the right-handed α-helical TRP, a strong positive peak around 230 nm was found in YYACAYY peptides, which corresponds to the other π–π* transition of phenolic side chain ( Supplementary Fig. 28 ). In the case of TRP with a right-handed α-helical conformation, these strong positive peaks at 200 nm and at 230 nm from π–π* transitions of tyrosine side chains are overlapped with the negative broad peaks centred around 208 nm from the π–π* transition and around 220 nm from the n–π* transition of the α-helical peptide bonds, resulting in a relatively weak negative peak at 217 nm, instead of showing two minima at 208 and 222 nm (refs 51 , 52 , 53 , 54 ) Noticeably, the dimer peptide exhibited a clear negative peak at 217 nm, which is known to be the characteristics of the right-handed α-helical structure for TRP, while a peak at 217 nm of monomer peptide was positive ( Supplementary Fig. 28 ). The result implies that the monomer has much less amount of α-helical structure compared with dimer peptide. Both NMR and CD analysis showed that the dimer YYACAYY peptide has a stable right-handed α-helical structure. Assembly mechanism The importance of tyrosine groups for the assembly can be confirmed by the experiment with other sequences. When each of the four tyrosine positions was replaced with a single alanine, these YYACAYA, YYACAAY, YAACAYY and AYACAYY sequences could not form facets. These results suggest that all four tyrosine groups in YYACAYY are involved in film growth. In addition, we observed that YYCYY, YYYCYYY, YYAACAAYY, YYGCGYY and YFCFY induced facet formation. When we replaced tyrosine with phenylalanine at the terminal position of the peptides, such as in FYCYF and FFCFF, the kinetic activity of faceting was inhibited ( Table 1 ). Interestingly, adding just one tyrosine residue to both ends (YYYCYYY) resulted in wrinkled multiple facets ( Supplementary Fig. 29 ). Indeed, aromatic–aromatic interaction between tyrosine groups can be frequently found in many natural proteins, where the distance between two ring centroids is between 4 and 7 Å (ref. 55 ). It is worthwhile to mention that the preferred geometry of two tyrosine groups can vary depending on the hydration of -OH group, which is influenced by the environment [56] . This influence is especially prominent when in a relatively hydrophobic region, such as an air/water interface and lipid membrane, or when exposed to the organic solvent, where the aromatic interactions between two tyrosine residues become more dominant than a possible hydrogen bonding with -OH. The interactions of peptides at the air/water interface during the peptide assembly was monitored by measuring the surface pressure change using the Wilhelmy plate method ( Supplementary Fig. 30 ). As expected, the surface pressure increased during the peptide assembly at the interface, with a faster increase at higher peptide concentration ( Supplementary Fig. 31a ), and with a maximum value at pH 6 ( Supplementary Fig. 31b ), which indicates the higher tendency of the peptide film assembly under those conditions. However, in the case of the YY and YYAKAYY peptides, the surface pressure increased only slightly ( Supplementary Fig. 32 ). In addition, a pressure change versus peptide concentration plot was analysed to estimate the standard Gibbs free energy of adsorption of the YYACAYY peptides at the interface and the intermolecular interaction energy ( Fig. 2c ). On the basis of assumption that the film thickening contributed marginally to the increase of surface pressure, we applied the Langmuir and the Frumkin isotherm models to our experimental data, which is described in detail in the Supplementary Note 2 . While the Langmuir isotherm model failed to explain the trend of the data, the close fit of the data to the Frumkin isotherm model shows that there is an attractive interaction among peptides, as verified by the negative Frumkin interaction factor. The calculated values of the standard Gibbs free energy of adsorption in the Langmuir and Frumkin isotherm model were −4.1 and −5.4 kcal mol −1 , respectively. Considering all the experimental data, we proposed the following mechanism of facet formation. YYACAYY is solubilized as a monomer without forming disulphide bonds. YYACAYY peptides adsorb on the air/water interface, and the anisotropic environment of the air/water interface can induce and further stabilize the specific peptide conformation by directing hydrophobic tyrosine regions into the air. As the local concentration increases at the interface, a lateral association begins to occur through the aromatic interactions among the tyrosines. In case of droplet, peptide rafts form and curvature induce migration of these rafts initiate the thick film formation on the top of the droplet. Simultaneously, peptides that are organized into a monolayer or raft form disulphide bonds and construct a thin nanosheet and the relatively oxygen-rich environment at the interface facilitates disulphide bond formation. Indeed, a sulfhydryl (-SH) group, which is not very active at a pH of 5, can be crosslinked by a disulphide bridge at the interface as a result of the proximity effect and the oxidative environment [57] . This dimerization stabilize the backbone conformation that facilitate the interaction between tyrosine groups vertically and laterally. This repeated dimerization and stacking results in the growth of the film and leads to the propagation of faceting. Applications to a bio-inspired catalytic scaffold One potential application of tyrosine containing peptide film is to serve as a redox-active scaffold for developing an enzyme mimetic catalyst. Here we explored the possibility of whether tyrosine radicals generated in our peptide film were able to trigger or enhance the chemical reaction in a manner similar to that observed for various biological systems. Tyrosyl radical generation is a key process for efficient electron transfer, as shown in photosystem II. Tyrosyl radicals can also cooperate with a neighbouring cysteine, as exemplified by ribonucleotide reductase and galactose oxidase. A class I ribonucleotide reductase produces sequential radicals of multiple tyrosine groups with Mn(IV) or Fe(IV) ions [58] and oxidizes cysteine residues, generating a sulfhydryl radical [59] to reduce deoxyribonucleotides to ribonucleotides. Galactose oxidase converts primary alcohols to aldehydes via a tyrosyl radical (Y·) generated by a Cu(II) ion [60] , [61] with the reduction of oxygen to hydrogen peroxide [62] . Despite the biological significance of tyrosine in proteins, the application of a tyrosyl radical in material synthesis has been limited, probably because monomeric tyrosyl radicals can be easily quenched in the reaction media, thus making the well-defined macroscopic structure difficult to obtain. Therefore, we expected our peptide film to be a unique platform, as it is based on a tyrosine-based platform that allows easy interfacing with any underlying electrode and systematic study of the ordering and neighbouring sequence effect. In fact, the cyclic voltammetry curve ( Fig. 5a ) indicates that tyrosyl radicals can be easily generated from our peptide film by applying a potential of 0.9 V versus the normal hydrogen electrode (NHE). 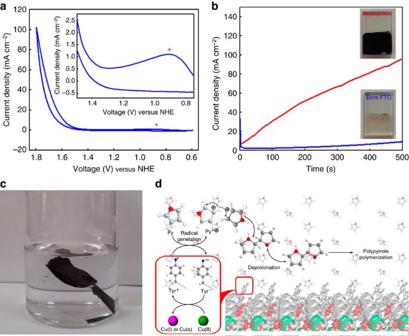Figure 5: Galvanostatic or Cu(II)-induced generation of tyrosyl radicals in peptide film. (a) Cyclic voltammetry (CV) polarization curve for the YYACAYY film on FTO glass in 0.1 M NaCl electrolyte. Electrochemical oxidation of tyrosine (Tyr→Tyr·) resulted in a broad peak (*), with the maximum current at 0.9 V (versus NHE). (b) The current density profiles of the YYACAYY peptide film (red) and tyrosine monomer (blue) deposited in FTO substrates during bulk electrolysis at 0.9 V in 0.1 M NaCl containing 50 mM pyrrole. After 30 min of electrolysis, remarkably different kinetics in polypyrrole formation could be confirmed by the colour change on the substrate (inset). (c) Photograph of the polypyrrole/peptide film suspended stably in neutral water. The peptide film assembled on the surface of water containing 4 mM CuCl2was able to induce the polymerization of pyrrole. (d) The schematics of the proposed mechanism involving Cu(II) reduction, tyrosyl radical generation and pyrrole oxidation. The Cu(II) reduction in distilled water spontaneously induced the formation of tyrosyl radical (Tyr·) without any additional oxidant or applied potential. Thereafter, the Tyr· initiates pyrrole polymerization. Figure 5: Galvanostatic or Cu(II)-induced generation of tyrosyl radicals in peptide film. ( a ) Cyclic voltammetry (CV) polarization curve for the YYACAYY film on FTO glass in 0.1 M NaCl electrolyte. Electrochemical oxidation of tyrosine (Tyr→Tyr·) resulted in a broad peak (*), with the maximum current at 0.9 V (versus NHE). ( b ) The current density profiles of the YYACAYY peptide film (red) and tyrosine monomer (blue) deposited in FTO substrates during bulk electrolysis at 0.9 V in 0.1 M NaCl containing 50 mM pyrrole. After 30 min of electrolysis, remarkably different kinetics in polypyrrole formation could be confirmed by the colour change on the substrate (inset). ( c ) Photograph of the polypyrrole/peptide film suspended stably in neutral water. The peptide film assembled on the surface of water containing 4 mM CuCl 2 was able to induce the polymerization of pyrrole. ( d ) The schematics of the proposed mechanism involving Cu(II) reduction, tyrosyl radical generation and pyrrole oxidation. The Cu(II) reduction in distilled water spontaneously induced the formation of tyrosyl radical (Tyr·) without any additional oxidant or applied potential. Thereafter, the Tyr· initiates pyrrole polymerization. Full size image To explore the possibility of using tyrosyl radicals in the film, we chose oxidative polymerization of pyrrole as a model reaction. In general, polypyrrole can be synthesized by applying a potential greater than 1.0 V or by using an oxidant, such as Fe(III) ions. Although polymerization can be initiated at ~0.9 V, according to previous reports [63] , the rate at this potential is too slow to obtain macroscopic polypyrrole deposition. Indeed, as shown in blue ( Fig. 5b and the corresponding inset), our experimental results also confirmed that 0.9 V bulk electrolysis produced a negligible amount of polypyrrole deposition on a fluorine-doped tin oxide (FTO) substrate. In contrast, when a constant potential of 0.9 V was applied to the YYACAYY film on the FTO, the current density drastically increased to 68 μA after 300 s and the black polypyrrole film was deposited continuously. Moreover, the YYACAYY peptide film on the FTO substrate was able to mediate the electron transfer from the pyrrole to the electrode and to lower the energy barrier for oxidative polymerization. On the basis of our study on the electrochemically driven tyrosyl radical generation, we designed an experiment to further mimic an enzyme, such as the above-mentioned galactose oxidase, in which the radical is generated by a valence change of the copper ion without applying any additional potential. We found significantly different activities of copper ions to oxidize pyrrole into polypyrrole in the presence of the YYACAYY film. For the experiment, a peptide film was assembled with a 4-mM Cu(II) chloride solution and then exposed to pyrrole vapour. A black polypyrrole film gradually formed on top of the peptide film, and after an overnight reaction, a free-standing hybrid film of polypyrroles and peptides was obtained ( Fig. 5c ). In contrast, neither Cu(II) chloride solution nor Cu(II) chloride with tyrosine monomer produced a polypyrrole film, even after a few days. These results show that the YYACAYY film allows the Cu(II) ions to oxidize pyrrole, probably by electron transfer mediated by tyrosyl radicals ( Fig. 5d ). The fact that the polypyrrole film formed only at the air/peptide interface also supports the observation that electrons are transferred from vapourized pyrroles to Cu(II) in solution through the YYACAYY film. We believe that the catalytic activity and selectivity can be further improved by the combination of the sequence design and structural alternations based on the YYACAYY platform. The advantage of this approach is that our peptide film formation can provide a platform for the construction of functionally controllable 2D nanostructures. The sequence-dependent self-assembly presented here highlights the role of peptide folding in molecular packing and the importance of specific amino acids in organization behaviours. Our findings provide new insight into self-assembled peptide interfaces through dynamic curvature control and site-selective functionalization. Furthermore, we expect that the unique biological roles of the tyrosine groups in enzymes, photoactive proteins and protein crosslinking can be applied in the development of peptide-based bio/electronic materials. The scalable and functionally extendable peptide surface could be utilized in many applications, floating scaffolds for cell culture, responsive vesicles for drug delivery, ion-selective membranes, 2D-ordered conducting polymers, elastic protein mimetics and tyrosine-based catalysts. Materials 2-Chlorotrityl chloride (CTC; 100–200 mesh, 1.26 mmol g −1 ) resin, filtered polypropylene reactors (Libra tube RT-20M, 20 ml), 2-(1H-benzotriazole-1-yl)-1,1,3,3-tetramethyluronium hexafluorophosphate, hydroxybenzotriazole and Fmoc-protected amino acids were purchased from BeadTech (Seoul, Korea). N,N -Diisopropylethylamine, triisopropylsilane, 3,6-dioxa-1,8-octanedithiol, 4-(3,6-dimethyl-1,3-benzothiazol-3-ium-2-yl)- N,N -dimethylaniline chloride (thioflavin-T), β-mercaptoethanol, HEPES buffer, uranyl acetate, anisole and trifluoroethanol were purchased from Aldrich (St Louis, MO, USA). Dichloromethane (DCM), N,N -dimethylformamide (DMF), methanol, piperidine, diethyl ether and trifluoroacetic acid (TFA), sodium hydroxide and hydrochloric acid were obtained from Dae-Jung Chemicals (Korea). Hydrogen peroxide (30%) was purchased from Junsei (Japan). Peptide synthesis The peptides were synthesized on a CTC resin (1.26 mmol g −1 ) with Fmoc/tBu chemistry in the filtered reactor. After loading the first amino acid (0.3~0.5 mmol g −1 ), each coupling step was performed with 2 eq. of Fmoc-amino acid, 2 eq. of 2-(1H-benzotriazole-1-yl)-1,1,3,3-tetramethyluronium hexafluorophosphate, 2 eq. of hydroxybenzotriazole and 4 eq. of N,N -diisopropylethylamine for 2 h until the Kaiser test was turned out negative. DCM and DMF in a ratio of 1:1 was used as a solvent. The deprotection step of Fmoc group proceeded for 20 min by 20% piperidine/DMF. Cleavage of the final peptides from the CTC resin was conducted in 93% TFA, 2% triisopropylsilane, 2% 3,6-dioxa-1,8-octanedithiol and 3% anisole for 90 min. The cleavage mixture was filtered and washed with DCM and methanol, and the filtrate was concentrated in vacuum. The resulting residue was precipitated with cold diethyl ether, centrifuged and dried in vacuum. The peptides were purified with reverse-phase HPLC, when necessary, and identified by MALDI–time-of-flight and ESI mass spectrometer. The purity of all the peptides was above 95%. Facet formation To identify the key amino acids in facet formation, a number of peptide sequences were synthesized, as shown in Supplementary Table 4 . The conditions for facet formation were tested by varying the dissolution method, temperature, pH, drop size of peptide solution and peptide concentration. The most effective conditions were chosen based on these preliminary experiments. Typically, the peptide was completely dissolved in 50 mM HEPES (pH 7.4) by briefly sonicating for 10 min and was then heated at 90 °C for 30 min in a closed system. The 30-min heating at 90 °C helped to achieve complete dissolution of peptides in the aqueous solution. An aliquot (100 μl) of the peptide solution was placed on a surface of siliconized glass (Hampton Research, HR3-231) using a pipette. Facet formation was observed with a droplet size up to 1 ml, but the maximum volume limit was not identified. When the peptide solution was placed in a Petri dish, a large film formed at the air/water interface, eventually fully covering the interface. The diameter of the largest films that we observed was 10 cm. Faceting took place along with film formation at peptide concentrations higher than 0.33 mM (0.3 mg ml −1 ). No faceting was observed below concentrations of 0.33 mM. Faceting was observed over a wide pH range (between 3 and 8). Atomic force microscopy A drop of peptide solution was placed on a siliconized glass, and was incubated for 30 min at room temperature to make a facet at water/air interface. The planar part at the top of the droplet was transferred onto a clean silicon wafer or a mica surface. The samples adsorbed on the surface were washed with distillated water to remove salt, and then were air dried for 10 min. AFM images were obtained with Dimension 3,100 (Veeco Instruments, Woodbury, NY) in tapping mode. Measurements were carried out using silicon cantilevers with a spring constant of 21–78 N m −1 (Nanoscience) and the resonance frequency of 260–410 kHz. The operating conditions for AFM were 0.5 Hz of scan rate. Transmission electron microscope Aliquot (20 μl) of the film containing mixture was deposited on a carbon-coated copper grid (200 mesh) and air dried for 5 min. The remaining liquid was removed with filter paper. For negative staining, the peptide was stained with 2% aqueous uranyl acetate (Electron Microscopy Sciences) that was centrifuged at 13,200 r.p.m. for 2 min. Then, the remaining staining solution was also removed with filter paper. The prepared TEM grids were kept in a desiccator before TEM imaging to ensure the removal of moisture. Then, the microscopic images were observed at 80 kV using a JEOL JEM-1010 TEM. Fluorescence imaging The peptide film was stained with thioflavin-T. The peptide (2.2 mM) was dissolved at 90 °C for 30 min in 20 mM HEPES buffer (pH 7.4) containing 250 μM thioflavin-T. Aliquot (100 μl) of the solution was dropped onto a siliconized glass and was air dried for 2 h to induce the film formation. After the facet was transferred onto a precleaned microscope slide, the sample was covered with a coverslip and the remaining solution was removed by using a filter paper. The dye-bound peptide film was subjected to fluorescence imaging analysis at 470±30 nm with excitation at 430±10 nm. The fluorescence images were obtained by using a Deltavision RT (AppliedPrecision, USA) microscope with an Olympus IX70 camera. Surface tension analysis The peptide was completely dissolved in distilled water by sonicating for 30 min at room temperature and heating at 90 °C for 30 min in a closed system. The peptide solution (10 ml) was carefully transferred into a Petri dish (60 × 15 mm 2 ), and the Wilhelmy plate was placed at the air/water interface. Then, the surface pressure changes were continuously monitored without compression at room temperature and 30±5% humidity. After the peptide solutions were exposed to air, the surface pressure increase over time was recorded ( Supplementary Fig. 13 ). The surface pressure time isotherm of YYACAYY was analysed at different peptide concentrations. FE simulation for real image-based geometry To calculate the deformed shape of the peptide film on the droplet in more detail, the real geometry of the peptide film on the droplet should be considered. The commercial software ABAQUS was used for the FE analysis. MALDI–time-of-flight mass spectrometry The matrix solution was prepared by dissolving 10 mg of 2,5-dihydroxy benzoic acid in 1 ml of a 3:7 mixture of deionized water and acetonitrile containing 0.1% TFA. Then, an aliquot (0.5 μl) of peptide solution or peptide films was dried, incubated with 0.5 μl of 20 mM DTT and treated with 8 mM of aqueous NH 3 for 5 min. The reaction was quenched by adding 0.5 μl of the matrix solution. All data were acquired with an Autoflex MALDI–TOF mass spectrometer (Bruker Daltonics) equipped with a Smartbeam laser controlled by FlexControl software (Bruker Daltonics). Mass spectra were acquired in the positive reflector mode using a 140-ns pulsed ion extraction and 1,000 mV digitizer sensitivity. ESI–mass spectrometry The peptide film was dissolved in 0.5% acetic acid/methanol. Mass data were confirmed by the analytical HPLC–ESI–mass spectrometer (MS; Thermo—Finnigan LCQ deca XP MS ESI–MS) and Phenomenex C4 reverse-phase column (4 μm, 100 × 3 mm 2 ). The gradient was 10–65% acetonitrile in H 2 O with 0.5% formic acid over 21 min. XRD analysis The XRD data were measured over the scattering angle ranging from 3° to 60° at 2 θ step of 0.02° using CuK α radiation with a secondary graphite monochromator in the reflection geometry at room temperature (Rigaku, D/max2200VK). Si (NIST SRM 640c) powder was used as an external standard to correct the zero-point shift for the measured diffraction data. FT-IR spectroscopy FT-IR spectra of YYACAYY (monomer or peptide films) were analysed with a Thermo Nicolet 6,700 FT-IR spectrometer equipped with an attenuated total reflection accessory. The film on the droplet was transferred to a clean silicon wafer, air dried for 24 h and placed on a ZnSe/diamond. The peptide film from a single batch gave an insufficient signal and, thus, films from 12 batches under the same conditions were transferred to the same silicon wafer for analysis. The scanned wave numbers ranged from 300 to 4,000 cm −1 at a resolution of 1.93 cm −1 . The spectra were scanned eight times. Raman spectroscopy Raman spectra of YYACAYY (monomer or peptide films) were analysed with Horiba Jobin–Yvon/LabRam Aramis Raman spectrometer (diode laser 785 nm, power=1 mW). The film on the droplet was transferred onto a clean gold-coated silicon wafer and air dried for 24 h. The single transfer of film did not give significant signals. Therefore, multiple transfers of the films were necessary on the substrate. The scanned wave numbers ranged between 200 and 3,000 cm −1 with 300 s scanning in average. Zeta potential measurement The surface charge of YYACAYY in aqueous solution was measured with Malvern Zetasizer, (Model Nano ZS, Malvern Instruments Ltd., UK) with a He-Ne (633 nM) laser (4.0 mW). The zeta potential data were collected with an Avalanche photodiode with QE >50% at 633 nM using the M3-PALS measurement technique. Supplementary Figure 5 shows the zeta potential–pH dependence curve of the peptide. NMR spectroscopy The YYACAYY peptide was dissolved at 3.0 mM in 0.45 ml of DMSO- d 6 (Cambridge Isotope Laboratories, Andover, MA, USA). Phase-sensitive 2D experiments were performed including double quantum-filtered correlation spectroscopy, total correlation spectroscopy (TOCSY) and NOE spectroscopy (NOESY), using 2D phase incrementation [64] , [65] , [66] , [67] . For the TOCSY and NOESY experiments, 350 transients with 2 K complex data points were collected at each increment with a relaxation delay of 1.5 s between successive transients. TOCSY experiments were performed using 60 and 80 ms MLEV-17 spin lock mixing pulses. Mixing times of 250 and 450 ms were used for NOESY experiments. For double quantum-filtered correlation spectroscopy experiments, 500 transients with 2 K complex data points were collected at each increment. The data along the t 1 dimension were zero-filled to 4 K before 2D Fourier transformation. To investigate the intramolecular hydrogen bondings in the peptide, the D 2 O exchange experiments were performed and the temperature coefficients of the amide protons were calculated by the use of the TOCSY experiments at 298, 303, 308, 313, 318, 323 and 333 K. All NMR spectra were recorded on a Bruker Avance 500, 700 and 800 MHz spectrometer at the Korea Basic Science Institute. NMR spectra were processed with NMRPipe [68] and visualized with Sparky [69] . CD spectroscopy The CD spectra of the 100-μM dimer peptide and 200 μM monomer peptides in 5 mM HEPES buffer at pH 7.4 were recorded using a J-810 spectropolarimeter (Jasco, Tokyo, Japan). The data from 10 scans were averaged for each spectrum. (Condition: 25 °C, 0.1 nm intervals, 190–300 nm, 1 mm path-length cell). How to cite this article: Jang, H.-S. et al . Tyrosine-mediated two-dimensional peptide assembly and its role as a bio-inspired catalytic scaffold. Nat. Commun. 5:3665 doi: 10.1038/ncomms4665 (2014).